Rapid changes in the electrical state of the 1999 Izmit earthquake rupture zone Crustal fluids exist near fault zones, but their relation to the processes that generate earthquakes, including slow-slip events, is unclear. Fault-zone fluids are characterized by low electrical resistivity. Here we investigate the time-dependent crustal resistivity in the rupture area of the 1999 M w 7.6 Izmit earthquake using electromagnetic data acquired at four sites before and after the earthquake. Most estimates of apparent resistivity in the frequency range of 0.05 to 2.0 Hz show abrupt co-seismic decreases on the order of tens of per cent. Data acquired at two sites 1 month after the Izmit earthquake indicate that the resistivity had already returned to pre-seismic levels. We interpret such changes as the pressure-induced transition between isolated and interconnected fluids. Some data show pre-seismic changes and this suggests that the transition is associated with foreshocks and slow-slip events before large earthquakes. Crustal structure in the fault zones is often characterized by low resistivity [1] , [2] , [3] , [4] , [5] , [6] , [7] , [8] , [9] , [10] , [11] , [12] , [13] , [14] , [15] , [16] , [17] , [18] , [19] , [20] , [21] , [22] , [23] that indicates crustal fluid and suggests a possible relation to earthquake generation. The North Anatolian Fault zone (NAFZ), northwestern Turkey, is characterized by the low resistivity structure and electromagnetic studies there are expected to provide important information on the relation of crustal fluid to earthquake generation. When the M w 7.6 Izmit earthquake occurred on 17 August 1999 along the NAFZ, five magnetotelluric (MT) sites (four along a profile crossing the NAFZ and one at a remote reference site ~40 km south ( Fig. 1 )) were recording the electromagnetic field in the area [4] . Although these MT sites were aimed at investigating the resistivity structure of the NAFZ [4] , [9] , [10] , they provide an extremely rare opportunity for studying pre- and co-seismic electromagnetic phenomena. Our preliminary analyses [4] , however, have not provided clear examples of anomalous changes, except for those associated with seismic waves [24] that could be interpreted in terms of the seismic dynamo effect [25] . A seismological study [26] found small foreshocks at site UCG ( Fig. 1 ) that began ~40 min before the mainshock. The waveforms of these events were similar to the mainshock, suggesting that they occurred where the mainshock began. Inspired by this report, we examined our MT data and found that two foreshocks and the mainshock caused electromagnetic field disturbances at site 120, from which we determined arrival times for these earthquakes. The difference in arrival times between the largest foreshock and the mainshock was 1′45.3″, and the time difference between the second largest foreshock and the mainshock was 12′15.6″. Using seismic data [26] , these time differences are 1′45.2″ and 12′15.7″, respectively, which suggests that the foreshocks occurred at approximately the same location as the mainshock. Recent detailed analysis of seismic data [27] has shown that foreshocks and numerous smaller events can be interpreted as indicating a slow rupture leading to the mainshock, as may have occurred before the 2011 M w 9.0 Tohoku-Oki earthquake [28] . 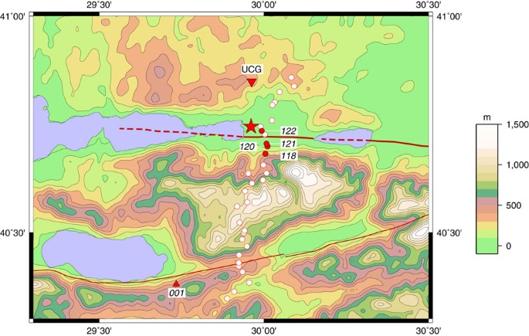Figure 1: Locations of sites. Sites 118, 120, 121, 122 and 001 (reference site). UCG is a seismic station at which foreshocks were observed26. Open circles indicate other sites where MT observations were made before and after the Izmit earthquake10, whose epicentre is shown by the red star31. The thick red line denotes the North Anatolian Fault, on which the rupture occurred. Figure 1: Locations of sites. Sites 118, 120, 121, 122 and 001 (reference site). UCG is a seismic station at which foreshocks were observed [26] . Open circles indicate other sites where MT observations were made before and after the Izmit earthquake [10] , whose epicentre is shown by the red star [31] . The thick red line denotes the North Anatolian Fault, on which the rupture occurred. Full size image In this study, we focus on the time variations of MT parameters, such as the apparent resistivity and impedance phase. However, the amount of data is not sufficient for this purpose; MT data sampled at 24 Hz are only available for 15 h, from 1700 to 0800 hours in local time, and for 7 days at site 118, 6 days at site 120, and 3 days at sites 121 and 122. However, continuous data are available for 10 h before the Izmit earthquake and 5 h after it. Similar data are also available at sites 121, 122 and 001 (the reference site) on 17 and 18 September, 1 month after the earthquake. These results show clear co-seismic and post-seismic changes in MT parameters. Co-seismic changes are characterized by abrupt decrease in crustal resistivity, while post-seismic changes suggest increase within 1 month. Some data indicate abrupt decrease in resistivity about 20 min before the mainshock. Two-dimensional (2D) models imply that the resistivity is decreased by 50–80% at 3–6 km depth. We interpret the abrupt changes in crustal resistivity found in association with the Izmit earthquake in terms of a transition from the state of isolated fluids to the state of interconnected fluids. Before the earthquake, some fluids are partially in an isolated state, and pore pressure change immediately before and during the earthquake connects the fluids through a new fluid-path network. Pre-seismic change suggests that the transition is associated with foreshocks and slow-slip events before the earthquake. 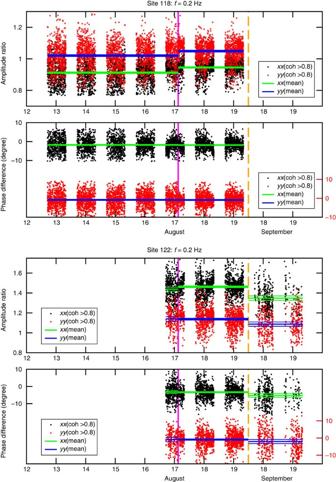Figure 2: Amplitude ratio of the horizontal magnetic field and phase difference. Estimates of the amplitude ratio of the horizontal magnetic field (H) at sites 118 and 122 relative to the reference site 001 are shown together with the associated phase difference at a frequency of 0.2 Hz. (xx) and (yy) correspond to the ratios ofHxandHy, respectively, at each site relative to the reference site.xis the northward component andyis the eastward component. The vertical axis for the phase for (yy) is given on the right side. Estimates with partial coherencies lower than the threshold value shown in the figure are excluded. The solid vertical line (purple) indicates the time of the mainshock. A 1-month gap in time is indicated by the dashed vertical line (orange). MT parameter estimates before and after the earthquake Figure 2 shows examples of the amplitude ratio of the horizontal magnetic field variation and the phase difference in the horizontal magnetic field derived from the diagonal elements of the transfer function matrix relating two components ( x : northward, y : eastward) of sites 118 and 122 relative to reference site 001 at a frequency of 0.2 Hz. Additional data are given in Supplementary Fig. S1 . Large fluctuations are due mostly to the inherently indeterminate nature of the two-input system with an imperfect independency between two inputs. In this article, we average all estimates before and after the Izmit earthquake to examine co-seismic changes. Error estimates of the mean value are discussed in the Methods section. Figure 2: Amplitude ratio of the horizontal magnetic field and phase difference. Estimates of the amplitude ratio of the horizontal magnetic field ( H ) at sites 118 and 122 relative to the reference site 001 are shown together with the associated phase difference at a frequency of 0.2 Hz. ( xx ) and ( yy ) correspond to the ratios of H x and H y , respectively, at each site relative to the reference site. x is the northward component and y is the eastward component. The vertical axis for the phase for ( yy ) is given on the right side. Estimates with partial coherencies lower than the threshold value shown in the figure are excluded. The solid vertical line (purple) indicates the time of the mainshock. A 1-month gap in time is indicated by the dashed vertical line (orange). 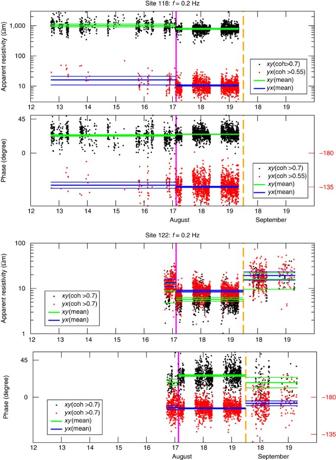Figure 3: Apparent resistivity and impedance phase. Estimates of the apparent resistivity are shown with impedance phase at sites 118 and 122 at a frequency of 0.2 Hz. (xy) corresponds to the pair ofEx(electric field) andHyat each site, and (yx) corresponds to the pair ofEy(electric field) andHxat each site. The vertical axis for the phase for (yx) is given on the right side. Estimates with partial coherencies lower than the threshold value shown in the figure are excluded. The solid vertical line (purple) indicates the time of the mainshock. A 1-month gap in time is indicated by the dashed vertical line (orange). Full size image Figure 3 shows examples of the apparent resistivity and impedance phase derived from the off-diagonal elements of the impedance tensor relating two components of the electrical field to two components of the horizontal magnetic field at sites 118 and 122. Again, we consider averages before and after the Izmit earthquake. Additional examples are given in Supplementary Fig. S2 . Figure 3: Apparent resistivity and impedance phase. Estimates of the apparent resistivity are shown with impedance phase at sites 118 and 122 at a frequency of 0.2 Hz. ( xy ) corresponds to the pair of E x (electric field) and H y at each site, and ( yx ) corresponds to the pair of E y (electric field) and H x at each site. The vertical axis for the phase for ( yx ) is given on the right side. Estimates with partial coherencies lower than the threshold value shown in the figure are excluded. The solid vertical line (purple) indicates the time of the mainshock. A 1-month gap in time is indicated by the dashed vertical line (orange). Full size image We question whether the observed changes in resistivity occurred in association with the foreshock cluster. Unfortunately, MT parameters are unlikely able to resolve such a short-term phenomenon. However, some results suggest possible changes during the foreshocks, as shown in Fig. 4 . If we focus on the foreshock activity, the apparent resistivity at site 122 at 0.2 Hz seems to have decreased ~20 min before the mainshock, while the apparent resistivity at 0.5 Hz changed at the time of the earthquake. A similar precursory change is also seen in the magnetic field amplitude ratio at site 118. Additional data are shown in Supplementary Figs S3,S4 . 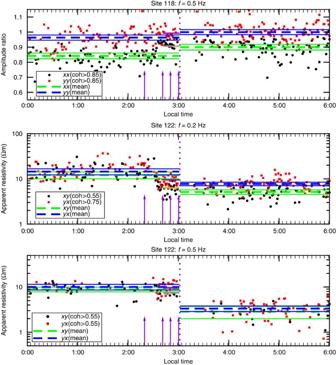Figure 4: MT parameters immediately before and after the earthquake. Estimates of the amplitude ratio for the horizontal magnetic field at site 118 at a frequency of 0.5 Hz and the apparent resistivity at site 122 at frequencies of 0.2 and 0.5 Hz are shown. Here the estimates over 6 h, including the mainshock, which is indicated by the dotted vertical line (purple), are only shown. The left three arrows correspond to the first, second and third pairs of foreshocks, and the right-most arrow indicates the largest foreshock. The short horizontal bars (orange and purple) denote the mean values for 20 min before the mainshock. In the first and second figures, the changes seem to have started ~20 min before the mainshock, whereas no pre-seismic change is seen in the third figure. Estimates with partial coherencies lower than the threshold coherency shown in each figure are excluded. Figure 4: MT parameters immediately before and after the earthquake. Estimates of the amplitude ratio for the horizontal magnetic field at site 118 at a frequency of 0.5 Hz and the apparent resistivity at site 122 at frequencies of 0.2 and 0.5 Hz are shown. Here the estimates over 6 h, including the mainshock, which is indicated by the dotted vertical line (purple), are only shown. The left three arrows correspond to the first, second and third pairs of foreshocks, and the right-most arrow indicates the largest foreshock. The short horizontal bars (orange and purple) denote the mean values for 20 min before the mainshock. In the first and second figures, the changes seem to have started ~20 min before the mainshock, whereas no pre-seismic change is seen in the third figure. Estimates with partial coherencies lower than the threshold coherency shown in each figure are excluded. 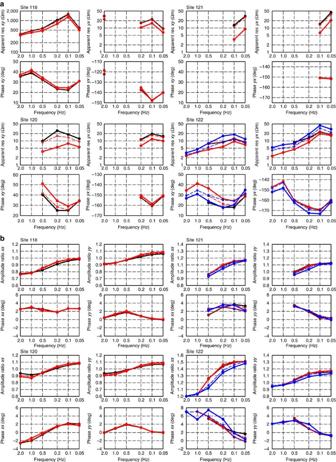Figure 5: Estimates before and after the earthquake. Estimates before the earthquake (black), immediately after the earthquake (solid red) and 1 month after the earthquake (solid blue) are shown for comparison. (a) Average apparent resistivity and impedance phase, and (b) average amplitude ratio and phase at six frequencies. Red and blue dots connected by dotted lines are estimates of the minimum changes. Full size image Figure 5a shows the co-seismic and post-seismic changes in the average apparent resistivity and impedance phase for each frequency at each site, together with the minimum changes in the confidence level, corresponding to ~99%. Many minimum changes are 0, which indicates no significant changes. Nearly all co-seismic changes are characterized by decreasing apparent resistivity, suggesting a temporary decrease in crustal resistivity. The post-seismic changes are characterized by increasing values, indicating recovery to the level before the earthquake. Figure 5: Estimates before and after the earthquake. Estimates before the earthquake (black), immediately after the earthquake (solid red) and 1 month after the earthquake (solid blue) are shown for comparison. ( a ) Average apparent resistivity and impedance phase, and ( b ) average amplitude ratio and phase at six frequencies. Red and blue dots connected by dotted lines are estimates of the minimum changes. Full size image Similarly, Fig. 5b shows the co-seismic and post-seismic changes in the average amplitude ratios and phase. Nearly all co-seismic changes are characterized by increasing amplitude ratio, again suggesting a temporary decrease in crustal resistivity. The post-seismic changes are characterized by decreasing values, again indicating recovery to the level before the earthquake. 2D models of resistivity structure To interpret the co-seismic changes in apparent resistivity and impedance phase, 2D models [4] , [9] , [10] derived from the 2D inversion code [29] for a long profile ( Fig. 1 ) are useful, and we modified these models along this profile ( Fig. 6a ). However, this 2D model is only an approximation of the actual complicated 3D structure. The estimated 2D strike based on the Groom and Baily decomposition [30] is ~50° East from North for frequencies lower than 0.1 Hz, reflecting a regional geological structure [10] , and it is nearly 90° for frequencies of 10–0.1 Hz, reflecting the local E–W fault structure. In this respect, the test model is more realistic for frequencies higher than 0.2 Hz. In this approximation, the components ( xx ) of the horizontal magnetic field ratio and phase and ( yx ) of the apparent resistivity and impedance phase correspond to the TE (transverse electric) mode. The components ( xy ) of apparent resistivity and impedance phase correspond to the TM (transverse magnetic) mode. For 2D models, no changes occur in the horizontal magnetic field for the TM mode. 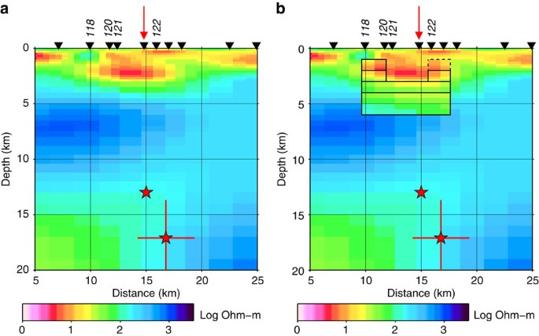Figure 6: Models of resistivity structure. (a) An initial test model derived from the regional two-dimensional model10. (b) A co-seismic model in which the resistivity in the area enclosed by the solid and dashed lines is decreased by 50% at 1–2 km depth, 10% at 2–3 km depth, by 50% at 3–4 km depth and by 80% at 4–6 km depth, compared with the initial resistivity model. A local pre-seismic model beneath site 122 corresponds to the co-seismic model without the shallow (1–2 km) zone denoted by the dashed rectangle. Figure 6: Models of resistivity structure. ( a ) An initial test model derived from the regional two-dimensional model [10] . ( b ) A co-seismic model in which the resistivity in the area enclosed by the solid and dashed lines is decreased by 50% at 1–2 km depth, 10% at 2–3 km depth, by 50% at 3–4 km depth and by 80% at 4–6 km depth, compared with the initial resistivity model. A local pre-seismic model beneath site 122 corresponds to the co-seismic model without the shallow (1–2 km) zone denoted by the dashed rectangle. Full size image As the co-seismic changes are largest at frequencies near 0.2 Hz, we presume a probable area of resistivity change as follows. A conductive zone with a resistivity of ~10 Ωm extends to a depth of 3 km, as shown in Fig. 6a , with a skin depth of ~3.5 km for 0.2 Hz. Below this conductive layer is a resistive zone on the order of 100 Ωm, with a skin depth of 10–20 km for 0.2 Hz. If the attenuation in the shallow conductive zone is considered, the penetration depth is likely to be shallower than 10 km. The horizontal extent is estimated as 6 km due to the large co-seismic changes observed at sites 120 and 122. Based on these considerations, we searched for a plausible model using the 2D forward-modelling code [29] . The models of the initial and co-seismic stages are shown in Fig. 6a . The pre-seismic model is uncertain due to a very limited data set, and it is supposed to be the same as the co-seismic stage except for a shallow layer between 1 and 2 km depth below site 122. This layer is not necessary to explain the pre-seismic change in apparent resistivity at site 122 observed at 0.2 Hz, but not at 0.5 Hz ( Fig. 4 ). However, it is necessary to explain the co-seismic change at 0.5 Hz. Addition of the second layer (2–3 km depth) better explains the observed results at site 122. The computed and observed changes in the apparent resistivity and impedance phase are shown in Fig. 7a and changes in the horizontal magnetic field amplitude ratio and phase are shown in Fig. 7b . 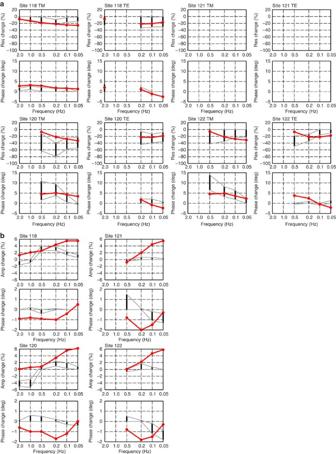Figure 7: Co-seismic changes at six frequencies. (a) Changes (black) in apparent resistivity (per cent) and impedance phase (degrees). (b) Changes (black) in amplitude ratio (per cent) and phase (degrees). Red dots show the estimates derived from the models shown inFig. 6. Figure 7: Co-seismic changes at six frequencies. ( a ) Changes (black) in apparent resistivity (per cent) and impedance phase (degrees). ( b ) Changes (black) in amplitude ratio (per cent) and phase (degrees). Red dots show the estimates derived from the models shown in Fig. 6 . Full size image Considering some ambiguities in the 2D approximation and errors in the observations, we conclude that these models can be used only to infer the possible location of an area of a resistivity anomaly and the magnitude of change. At 3–6 km depth, the resistivity is decreased by 50% in its shallow part (3–4 km) and by 80% in its deep part (4–6 km). Resistivity changes in additional local layers are 10% for 2–3 km and 50% for 1–2 km. This depth range is shallower than the hypocentre of the mainshock, which is estimated to be 10–15 km (refs 26 , 31 ), but it is consistent with the distribution of major fault slip during the Izmit earthquake [32] . We conclude that a co-seismic change in crustal resistivity occurred. Conventionally, crustal resistivity is thought to change gradually, reflecting the diffusion of fluid as in a classical dilatancy diffusion model [33] . We propose an alternative model: a transition from the state of isolated fluids to the state of interconnected fluids. The crustal resistivity is primarily controlled by conductive crustal fluid and its interconnectivity at the microscopic level, such as on grain boundaries or along micro-cracks [34] , [35] , [36] , [37] , [38] , [39] . Our conceptual model is as follows: before the earthquake, some fluids were partially in an isolated state, and the pore pressure changed immediately before and during the earthquake, connecting the fluids through a new fluid-path network. In this respect, the role of crustal fluids in the triggering of earthquakes has been discussed previously [40] , [41] , [42] , and we propose that this transition may be triggered by the release of stress due to slow slip at the rupture initiation zone and during the earthquake rupture. The opposite can be considered for a possible relation to the slow slip; coupling at the fault interface is weakened by the fluid-filled network that is created by the increase in pressure, which results in increased fault slip. The post-seismic restoration to the pre-seismic level over 1 month seems to be consistent with the post-seismic crustal deformation after the mainshock [43] , although no MT data are available between 20 August and 17 September. We need more examples of the changes in crustal resistivity associated with earthquakes, but we believe that variations in the electrical state are related actively or passively to the generation of earthquakes. Our model suggests that in future studies, more attention should be paid to the areas of intermediate resistivity (~100 Ωm), where the partial interconnection of fluids is expected; in low-resistivity areas, the fluid network is nearly complete and in high-resistivity areas, the amount of fluid is insufficient for effective fluid interconnectivity. In fact, earthquakes tend to occur at boundaries between high- and low-resistivity areas [4] , [6] , [7] , [9] , [22] . MT parameter estimation for available data To focus on the slow rupture process over the course of tens of minutes, we computed MT parameters at 1-min intervals. The sampling rate is 24 Hz, resulting in 1,440 data points for 1 min of data. This limits the lower-frequency range to ~0.05 Hz; hence, we examined MT parameters for six frequencies: 0.05, 0.1, 0.2, 0.5, 1.0 and 2.0 Hz. We used a conventional spectral analysis based on the Fourier transformation of auto- and cross-correlation functions. According to our preliminary spectral analysis for the data set, the lower-frequency end for a specific lag provides more reliable spectral estimates mainly due to dominant power towards lower frequencies. Therefore, we made calculations by varying the lag for each of the six frequencies. This resulted in more reliable spectral estimates at higher frequencies than for fixed lags for all frequencies. Some of minute-long data include insufficient magnetic source signals, resulting in less-reliable estimates of MT parameters, but we omitted such data by setting a threshold to the partial coherency. A severe problem was noted during visual inspection of the time-series data: several large noise spikes that affect all frequency ranges. We therefore included an algorithm to automatically remove such noise in preprocessing, which improved the quality of the data. From spectral estimates, we computed the impedance tensor elements at each site. The transfer function matrix relating the two components of the magnetic field at each site to the reference site was also calculated. We refer to these as MT parameters. The main purpose of our electromagnetic observations was to reveal the MT-based resistivity structure along the north–south profile crossing the NAFZ. We typically occupied one site for a few days and moved to the next site using four sets of MT equipment (Phoenix system). Observations were made from 1700 to 0800 hours in local time (15 h total) to acquire higher-quality data during the night. When the Izmit earthquake occurred, sites 118, 120, 121, 122 and 001 (the reference site) were in operation, and we maintained these sites for 2 days after the earthquake. As a result, the observation periods are 7 days for site 118, 6 days for site 120 and 3 days for sites 121 and 122. One month later, we reoccupied sites 121, 122 and 001 for 2 days with the same equipment and observation configuration for each site, enabling us to examine possible post-seismic changes in MT parameters. During the observations, two components of the electric field and three components of the magnetic field were simultaneously measured at each site, including the remote reference site. The addition of the reference site is very important in our analyses. For example, the changes in MT parameters that are unrelated to possible changes in the crustal resistivity at sites near the seismic rupture zone can be estimated using the parameters at the reference site. Daily variations in the impedance and phase were noted at the reference site. We ascribe these variations to the temperature of the induction coil used for magnetic field measurements. We buried the coils at a few tens of centimetres depth, exposing them to temperature variations, particularly during the day. Taking the ratio of the magnetic field measured at a survey site and the reference site reduces this effect because the temperature effects are similar for coils of the same type. The impedance tensor is the ratio of the electric to magnetic fields, and it is affected by the temperature of the magnetic sensor coil. To eliminate this effect, the ratio of the apparent resistivities at the study and reference sites is taken, and the apparent resistivity averaged for all available data at the reference site is used to recover the apparent resistivity at the study site. Similarly, the difference between the phases at two sites is taken and the phase averaged for all available data at the reference site is used to recover the phase at the study site. Statistical significance During our analyses, we noted some outliers and set the following criterion to remove them. For each real and quadrature part of the impedance tensor element or transfer function matrix element, the mean ( m ) and the s.d. ( σ ) were calculated from the data set for a few days after the earthquake. Then, values beyond the range between m −3 σ and m +3 σ were excluded from the data set. The same criterion was also applied to phase estimates computed from the estimates of the real and quadrature parts. Last, we comment on the error estimate of the mean value. If fluctuations are regarded as random, the statistical confidence interval of the estimated mean value is given as ασn −1/2 , where n is the number of samples and σ is the s.d. with α describing the level of confidence. We usually consider an ~99% confidence interval and adopt α =3. As noted above, we should consider possible remaining effects of temperature, even though the temperature effects are removed by taking the ratio or differences using data recorded simultaneously at the reference site. This is why we chose α =4 for the amplitude ratio, the associated phase and the MT phase. For the apparent resistivity, α =8. We define this as the error for the mean values before and after the earthquake. We verified that with these criteria, most mean estimates of apparent resistivity and phase at the reference site are within the confidence limit. The more robust method would be to consider median values instead of mean values, and interquartile deviations instead of s.d. We compared these and found that the results based on the above procedure are still reasonable, although some improvements are seen in medians at low frequencies. How to cite this article: Honkura, Y. et al . Rapid changes in the electrical state of the 1999 Izmit earthquake rupture zone. Nat. Commun. 4:2116 doi: 10.1038/ncomms3116 (2013).